Germline variation at 8q24 and prostate cancer risk in men of European ancestry Chromosome 8q24 is a susceptibility locus for multiple cancers, including prostate cancer. Here we combine genetic data across the 8q24 susceptibility region from 71,535 prostate cancer cases and 52,935 controls of European ancestry to define the overall contribution of germline variation at 8q24 to prostate cancer risk. We identify 12 independent risk signals for prostate cancer ( p < 4.28 × 10 −15 ), including three risk variants that have yet to be reported. From a polygenic risk score (PRS) model, derived to assess the cumulative effect of risk variants at 8q24, men in the top 1% of the PRS have a 4-fold (95%CI = 3.62–4.40) greater risk compared to the population average. These 12 variants account for ~25% of what can be currently explained of the familial risk of prostate cancer by known genetic risk factors. These findings highlight the overwhelming contribution of germline variation at 8q24 on prostate cancer risk which has implications for population risk stratification. Prostate cancer (PCa) is the most common cancer among men in the US, with 161,360 new cases and 26,730 related deaths estimated in 2017 [1] . Familial and epidemiological studies have provided evidence of substantial heritability of PCa [2] , and ~170 common risk loci have been identified through genome-wide association studies (GWAS) [3] . The susceptibility region on chromosome 8q24 has been shown to be a major contributor to PCa risk, with multiple variants clustered in five linkage disequilibrium (LD) blocks spanning ~600 Mb that are independently associated with risk [4] . Many of these association signals reported at 8q24 have been replicated across racial/ethnic populations [5] , [6] , pointing to common shared functional variants within 8q24. However, rare ancestry-specific variants have also been detected, which confer larger relative risks of PCa (odds ratios [ORs] >2.0) than common risk variants in the region and signify allelic heterogeneity in the contribution of germline variation at 8q24 to PCa risk across populations [7] . In the current study, we perform a comprehensive investigation of genetic variation across the 1.4 Mb cancer susceptibility region at 8q24 (127.6–129.0 Mb) in relation to PCa risk. We combine genotyped and imputed data from two large GWAS consortia (PRACTICAL/ELLIPSE OncoArray and iCOGS) including >124,000 individuals of European ancestry to search for novel risk variants, as well as to determine the overall contribution of genetic variation at 8q24 to PCa heritability. Our findings underscore the sizable impact of genetic variation in the 8q24 region in explaining inter-individual differences in PCa risk, with potential clinical utility for genetic risk prediction. Marginal and conditional association analysis Genotype data from the Illumina OncoArray and iCOGS array and imputation to 1000 Genomes Project (1KGP) were generated among 71,535 PCa cases and 52,935 controls of European ancestry from 86 case-control studies (see Methods). Of the 5600 genotyped and imputed variants at 8q24 (127.6–129.0 Mb) with minor allele frequency (MAF) > 0.1% retained for analysis (see Methods), 1268 (23%) were associated with PCa risk at p < 5×10 −8 while 2772 (49%) were marginally associated at p < 0.05. These 5600 markers capture, at r 2 > 0.8, 90% and 97% of all variants at 8q24 (127.6–129.0 Mb) with MAF ≥ 1% and ≥5%, respectively (based on 1KGP Phase 3 EUR panel). 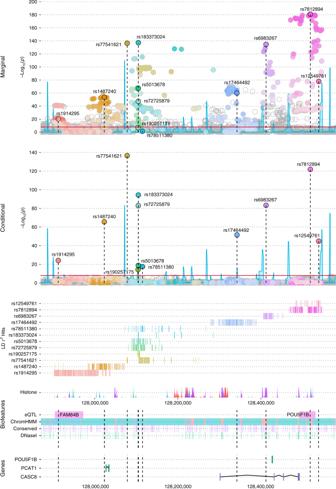Fig. 1 LocusExplorer plots of the 12 variants at 8q24 significantly associated with PCa risk. ‘Marginal’ and ‘Conditional’ Manhattan plot panels show marginal and conditional association results, respectively. Variant positions (x-axis) and −log10p-values from the Wald test (y-axis) are shown, with the red line indicating the threshold for genome-wide significant association with PCa risk (p≤ 5 × 10−8) and blue peaks local estimates of recombination rates. The position of the 12 independent variants is labeled in each plot. Clusters of correlated variants for each independent signal are distinguished using different colors and also depicted on the ‘LDr2Hits’ track. Stronger shading indicates greater correlation with the lead variant, with variants not correlated atr2≥ 0.2 with any lead variant uncolored. Pairwise correlations are based on the European ancestry (EUR) panel from the 1000 Genomes Project (1KGP) Phase 3. The relative position of RefSeq genes and biological annotations are shown in the ‘Genes’ and ‘Biofeatures’ panels, respectively. Genes on the positive strand are denoted in green and those on the negative strand in purple. Annotations displayed are: histone modifications in ENCODE tier 1 cell lines (Histone track), the positions of any variants that were eQTLs with prostate tumor expression in TCGA prostate adenocarcinoma samples and the respective genes for which expression is altered (eQTL track), chromatin state categorizations in the PrEC cell-line by ChromHMM (ChromHMM track), the position of conserved element peaks (Conserved track) and the position of DNaseI hypersensitivity site peaks in ENCODE prostate cell-lines (DNaseI track). The data displayed in this plot may be explored interactively through the LocusExplorer application (http://www.oncogenetics.icr.ac.uk/8q24/) In a forward and backward stepwise selection model on variants marginally associated with PCa risk ( p < 0.05, n = 2772; see Methods), we identified 12 variants with conditional p -values from the Wald test between 2.93 × 10 −137 and 4.28 × 10 −15 (Table 1 ). None of the other variants were statistically significant at p < 5 × 10 −8 after adjustment for the 12 independent hits (Fig. 1 ). The 8q24 region is shown in Supplementary Fig. 1 . Of these 12 stepwise signals, three had alleles with extreme risk allele frequencies (RAFs) that conveyed large effects (rs77541621, RAF = 2%, OR = 1.85, 95%CI = 1.76–1.94; rs183373024, RAF = 1%, OR = 2.67, 95%CI = 2.43–2.93; rs190257175, RAF = 99%, OR = 1.60, 95%CI = 1.42–1.80). The remaining variants had RAFs between 0.11 and 0.92 and conditional ORs that were more modest and ranged from 1.10 to 1.37 (Table 1 ). For 8 of the 12 variants, the allele found to be positively associated with PCa risk was the predominant allele (i.e., >50% in frequency). For two variants, rs78511380 and rs190257175, the marginal associations were not genome-wide significant and substantially weaker than those in the conditional model. For rs78511380, the marginal OR was slightly protective (OR = 0.97; p = 0.027), but reversed direction and was highly statistically significant when conditioning on the other 11 variants (OR = 1.19; p = 3.5 × 10 −18 ; Table 1 ). Table 1 Marginal and conditional estimates for genetic markers at 8q24 independently associated with prostate cancer risk Full size table Fig. 1 LocusExplorer plots of the 12 variants at 8q24 significantly associated with PCa risk. ‘Marginal’ and ‘Conditional’ Manhattan plot panels show marginal and conditional association results, respectively. Variant positions ( x -axis) and −log 10 p- values from the Wald test ( y -axis) are shown, with the red line indicating the threshold for genome-wide significant association with PCa risk ( p ≤ 5 × 10 −8 ) and blue peaks local estimates of recombination rates. The position of the 12 independent variants is labeled in each plot. Clusters of correlated variants for each independent signal are distinguished using different colors and also depicted on the ‘LD r 2 Hits’ track. Stronger shading indicates greater correlation with the lead variant, with variants not correlated at r 2 ≥ 0.2 with any lead variant uncolored. Pairwise correlations are based on the European ancestry (EUR) panel from the 1000 Genomes Project (1KGP) Phase 3. The relative position of RefSeq genes and biological annotations are shown in the ‘Genes’ and ‘Biofeatures’ panels, respectively. Genes on the positive strand are denoted in green and those on the negative strand in purple. Annotations displayed are: histone modifications in ENCODE tier 1 cell lines (Histone track), the positions of any variants that were eQTLs with prostate tumor expression in TCGA prostate adenocarcinoma samples and the respective genes for which expression is altered (eQTL track), chromatin state categorizations in the PrEC cell-line by ChromHMM (ChromHMM track), the position of conserved element peaks (Conserved track) and the position of DNaseI hypersensitivity site peaks in ENCODE prostate cell-lines (DNaseI track). The data displayed in this plot may be explored interactively through the LocusExplorer application ( http://www.oncogenetics.icr.ac.uk/8q24/ ) Full size image Haplotype analysis The haplotype analysis showed an additive effect of the 12 independent risk variants consistent with that predicted in the single variant test; co-occurrence of the 8q24 risk alleles on the same haplotype does not further increase the risk of PCa (Supplementary Table 1 ). The unique haplotype carrying the reference allele for rs190257175 (GCTTAT, 0.5% frequency) is also the sole haplotype associated with a reduced risk of PCa, suggesting that having the C allele confers a protective effect. The reference allele for rs78511380 (A, 8% frequency) occurs on a haplotype in block 2 together with the risk alleles for rs190257175, rs72725879 and rs5013678 (haplotype GTTTAA, 8%) which obscures the positive association with the T allele of rs78511380. Thus, the marginal protective effect associated with the risk allele for rs78511380 reflects an increased risk associated with the occurrence on a risk haplotype with other risk alleles (Supplementary Table 1 ). Correlation with known risk loci The 12 risk variants spanned across the five LD blocks previously reported to harbor risk variants for PCa at 8q24 [4] , with block 2 harboring six signals, blocks 1 and 5 two signals each, and blocks 3 and 4 only one (Supplementary Fig. 2 ). Except for a weak correlation between rs72725879 and rs78511380 in block 2 ( r 2 = 0.28), the risk variants were uncorrelated with each other ( r 2 ≤ 0.09; Supplementary Data 1 ), which corroborates their independent association with PCa risk. Eight of the variants (rs1487240, rs77541621, rs72725879, rs5013678, rs183373024, rs17464492, rs6983267, rs7812894) have been previously reported either directly (Supplementary Table 2 ) or are correlated ( r 2 ≥ 0.42) with known markers of PCa risk from studies in populations of European, African or Asian ancestry (Supplementary Data 1 ) [4] , [7] , [8] , [9] , [10] . The marginal estimates for previously published PCa risk variants at 8q24 in the current study are shown in Supplementary Table 2 . The variant rs1914295 in block 1 is only weakly correlated with the previously reported risk variants rs12543663 and rs10086908 ( r 2 = 0.17 and 0.14, respectively), while rs7851380 is modestly correlated with the previously reported risk variant rs1016343 ( r 2 = 0.28). The remaining two variants, rs190257175 and rs12549761, are not correlated ( r 2 < 0.027) with any known PCa risk marker. Polygenic risk score and familial relative risk To estimate the cumulative effect of germline variation at 8q24 on PCa risk, a polygenic risk score (PRS) was calculated for the 12 independent risk alleles from the final model based on allele dosages weighted by the per-allele conditionally adjusted ORs (see Methods). Compared to the men at ‘average risk’ (i.e., the 25th–75th PRS range among controls), men in the top 10% of the PRS distribution had a 1.93-fold relative risk (95%CI = 1.86–2.01) (Table 2 ), with the risk being 3.99-fold higher (95%CI = 3.62–4.40) for men in the top 1%. Risk estimates by PRS category were not modified by family history (FamHist-yes: OR = 4.24, 95%CI = 2.85–6.31; FamHist-no: OR = 3.38, 95%CI = 2.88–3.97). To quantify the impact of germline variation at 8q24, we also estimated the proportion of familial relative risk (FRR) and heritability of PCa contributed by 8q24 and compared this to the proportions explained by all known PCa risk variants including 8q24 (see Methods). The 175 established PCa susceptibility loci identified to date [3] , [11] are estimated to explain 37.08% (95%CI = 32.89–42.49) of the FRR of PCa, while the 12 independent signals at 8q24 alone capture 9.42% (95%CI = 8.22–10.88), which is 25.4% of the total FRR explained by known genetic risk factors for PCa (Table 3 ). This is similar to the proportion of heritability explained by 8q24 variants (22.2%) compared to the total explained heritability by the known risk variants (0.118). In comparison, the next highest contribution of an individual susceptibility region to the FRR of PCa is the TERT region at chromosome 5p15, where 5 independent signals contributed 2.63% (95%CI = 2.34–3.00). No other individual GWAS locus has been established as explaining >2% of the FRR, including the low frequency, non-synonymous, moderate penetrance HOXB13 variant (rs138213197) at chromosome 17q21 that is estimated to explain only 1.91% (95%CI = 1.20–2.85) of the FRR [11] . Table 2 Relative risk of PCa for polygenic risk score (PRS) groups Full size table Table 3 Proportion of familial relative risk (FRR) and heritability (h g 2 ) of PCa explained by known risk variants Full size table JAM analysis We explored our data with a second fine-mapping approach, JAM (Joint Analysis of Marginal summary statistics) [12] , which uses GWAS summary statistics to identify credible sets of variants that define the independent association signals in susceptibility regions (see Methods). The 95% credible set for the JAM analysis confirmed all of the independent signals from stepwise analysis except rs190257175, for which evidence for an association was weak (variant-specific Bayes factor (BF) = 1.17). There were 50 total variants included in the 95% credible set, and 174 after including variants in high LD ( r 2 > 0.9) with those in the credible set (Supplementary Data 2 ). In this large study of germline genetic variation across the 8q24 region, we identified 12 independent association signals among men of European ancestry, with three of the risk variants (rs1914295, rs190257175, and rs12549761) being weakly correlated ( r 2 ≤ 0.17) with known PCa risk markers. The combination of these 12 independent signals at 8q24 capture approximately one quarter of the total PCa FRR explained by known genetic risk factors, which is substantially greater than any other known PCa risk locus. The 8q24 region is the major susceptibility region for PCa; however, the underlying biological mechanism(s) through which germline variation in this region influences PCa risk remains uncertain. For each of the 12 risk variants at 8q24, the 95% credible set defined noteworthy (i.e., putative functional) variants based on summary statistics while accounting for LD. To inform biological functionality, we overlaid epigenetic functional annotation using publicly available datasets (see Methods) with the location of the 12 independent signals (and corresponding 174 variants within their 95% credible sets; Supplementary Data 3 ). Of the 12 independent lead variants, 6 are situated within putative transcriptional enhancers in prostate cell-lines; either through intersection with H3K27AC (rs72725879, rs5013678, rs78511380, rs6983267 and rs7812894) or through a ChromHMM enhancer annotation (rs17464492, rs6983267, rs7812894). Eight of the 12 stepwise hits (rs77541621, rs190257175, rs5013678, rs183373024, rs78511380, rs17464492, rs6983267, rs7812894) also intersect transcription factor binding site peaks from multiple ChIP-seq datasets representing the AR, ERG, FOXA1, GABPA, GATA2, HOXB13, and NKX3.1 transcription factors, with all 8 intersecting a FOXA1 mark and half an AR binding site. These variants may therefore exert their effect through regulation of enhancer activity and long-range expression of genes important for cancer tumorigenesis and/or progression [13] . The variant rs6983267 has also been shown to act in an allele-specific manner to regulate prostate enhancer activity and expression of the proto-oncogene MYC in vitro and in vivo [14] , [15] . However, despite the close proximity to the MYC locus, no direct association has been detected between 8q24 risk alleles and MYC expression in normal and tumor human prostate tissues [16] . The rare variant with the largest effect on risk, rs183373024, shows high evidence of functionality based on overlap with multiple DNaseI and transcription factor binding site peaks (for AR, FOXA1, HOXB13, and NKX3.1), which supports previous findings of an allele-dependent effect of this variant on the disruption of a FOXA1 binding motif [17] . Seven independent signals (rs1914295, rs1487240, rs77541621, rs72725879, rs5013678, rs183373024, rs78511380) and variants correlated at r 2 > 0.9 with these signals (Supplementary Data 2 ) are located within or near a number of prostate cancer–associated long noncoding RNAs (lncRNAs), including PRNCR1 , PCAT1 , and CCAT2 , previously reported to be upregulated in human PCa cells [18] and tissues [19] , [20] . Based on eQTL annotations in prostate adenocarcinoma cells, the independent signal rs1914295 and three correlated variants ( r 2 > 0.9; Supplementary Data 2 ) are associated with overexpression of FAM84B , a gene previously associated with progression and poor prognosis of PCa in animal studies [21] . Variants correlated at r 2 > 0.9 with rs7812894 ( n = 9; Supplemental Table 4 ) are eQTLs for POU5F1B , a gene overexpressed in cancer cell lines and cancer tissues [22] , [23] , although its role in PCa development is unknown. Whilst we have successfully refined the 8q24 region and identified a subset of variants with putative biological function within our credible set, multi-ethnic comparisons may help refine the association signals even further and precisely identify the functional alleles and biological mechanisms that modify PCa risk. Whereas the individual associations of the 8q24 variants with PCa risk are relatively modest (ORs < 2.0, except for rs183373024), their cumulative effects are substantial, with risk being 4-fold higher for men in the top 1% of the 8q24-only PRS. The contribution to the overall FRR of PCa is substantially greater for the 8q24 region (9.42%) than for any other known GWAS locus, including the moderate penetrance non-synonymous variant in HOXB13 (1.91%). The ability of these markers to explain ~25.4% of what can be currently explained by all known PCa risk variants is a clear indication of the important contribution of germline variation at 8q24 on PCa risk. Our study was predominantly powered to analyze variants with MAF > 1% as the imputed variants with MAF = 0.1-1% were most likely to fail quality control (QC); however, the high density of genotyped markers and haplotypes at 8q24 in the OncoArray and iCOGS studies provided a robust backbone for imputation and increased the chances to impute lower MAF variants with high imputation quality score. Understanding of the biology of these variants and the underlying genetic basis of PCa could provide new insights into the identification of reliable risk-prediction biomarkers for PCa, as well as enable the development of effective strategies for targeted screening and prevention. Study subjects, genotyping, and quality control We combined genotype data from the PRACTICAL/ELLIPSE OncoArray and iCOGS consortia [3] , [24] , which included 143,699 men of European ancestry from 86 case-control studies largely based in either the US or Europe. In each study, cases primarily included men with incident PCa while controls were men without a prior diagnosis of the disease. Both of the OncoArray and iCOGS custom arrays were designed to provide high coverage of common alleles (minor allele frequency [MAF] > 5%) across 8q24 (127.6–129.0 Mb) based on the 1000 Genomes Project (1KGP) Phase 3 for OncoArray, and the European ancestry (EUR) panel from HapMap Phase 2 for iCOGS. A total of 57,580 PCa cases and 37,927 controls of European ancestry were genotyped with the Illumina OncoArray, and 24,198 PCa cases and 23,994 controls of European ancestry were genotyped with the Illumina iCOGS array. For both studies, sample exclusion criteria included duplicate samples, first-degree relatives, samples with a call rate <95% or with extreme heterozygosity ( p < 10 −6 ), and samples with an estimated proportion of European ancestry <0.8 [3] , [24] . In total, genotype data for 53,449 PCa cases and 36,224 controls from OncoArray and 18,086 PCa cases and 16,711 controls from iCOGS were included in the analysis. Genetic variants with call rates <0.95, deviation from Hardy-Weinberg equilibrium ( p < 10 −7 in controls), and genotype discrepancy in >2% of duplicate samples were excluded. Of the final 498,417 genotyped variants on the OncoArray and 201,598 on the iCOGS array that passed QC, 1581 and 1737 within the 8q24 region, respectively, were retained for imputation. All studies complied with all relevant ethical regulations and were approved by the institutional review boards at each of the participating institutions. Informed consent was obtained from all study participants. Additional details of each study are provided in the Supplementary Note 1 . Imputation analysis Imputation of both OncoArray and iCOGS genotype data was performed using SHAPEIT [25] and IMPUTEv2 [26] to the October 2014 (Phase 3) release of the 1KGP reference panel. A total of 10,136 variants from OncoArray and 10,360 variants from iCOGS with MAF > 0.1% were imputed across the risk region at 8q24 (127.6-129.0 Mb). Variants with an imputation quality score >0.8 were retained for a total of 5600 overlapping variants between the two datasets. Statistical analysis Unconditional logistic regression was used to estimate per-allele odds ratios (ORs) and 95% confidence intervals (CIs) for the association between genetic variants (single nucleotide polymorphisms and insertion/deletion polymorphisms) and PCa risk adjusting for country and principal components (7 for OncoArray and 8 for iCOGS). Allele dosage effects were tested through a 1-degree of freedom two-tailed Wald trend test. The marginal risk estimates for the 5600 variants at 8q24 that passed QC were combined by a fixed effect meta-analysis with inverse variance weighting using METAL [27] . A modified forward and backward stepwise model selection with inclusion and exclusion criteria of p ≤ 5 × 10 −8 was performed on variants marginally associated with PCa risk from the meta results ( p < 0.05, n = 2772). At each step, the effect estimates for the candidate variants from both studies (OncoArray and iCOGS) were meta-analyzed and each variant was incorporated into the model based on the strength of association. All remaining variants were included one-at-a-time into the logistic regression model conditioning on those already incorporated in the model. We applied a conservative threshold for independent associations, with variants kept in the model if their meta p-value from the Wald test was genome-wide significant at p ≤ 5 × 10 −8 after adjustment for the other variants in the model. Correlations between variants in the final model and previously published PCa risk variants at 8q24 were estimated using the 1KGP Phase 3 EUR panel (Supplementary Data 1 ). Haplotype analysis Haplotypes were estimated in the Oncoarray data only using variants from the final stepwise model selection ( n = 12) and the EM algorithm [28] within LD block regions inferred based on recombination hotspots using Haploview 4.2 (Broad Institute, Cambridge, MA, USA) [29] . Only haplotypes with an estimated frequency ≥0.5% were tested. Polygenic risk score and familial relative risk An 8q24-only polygenic risk score (PRS) was calculated for variants from the final model ( n = 12) with allele dosage from OncoArray and iCOGS weighted by the per-allele conditionally adjusted ORs from the meta-analysis. Categorization of the PRS was based on the percentile distribution in controls, and the risk for each category was estimated relative to the interquartile range (25–75%) in OncoArray and iCOGS separately, and then meta-analyzed across the two studies. We estimated the contribution of 8q24 variants to the familial (first-degree) relative risk (FRR) of PCa (FRR = 2.5) [30] under a multiplicative model, and compared this to the FRR explained by all known PCa risk variants including 8q24 (Supplementary Data 4 ). We also estimated heritability of PCa using the LMM approach as implemented in GCTA [31] . For regions which have been fine-mapped using the OncoArray meta-analysis data, we used the updated representative lead variants, otherwise the originally reported variant was included provided that it had replicated at genome-wide significance in the meta-analysis; this identified a total of 175 independently associated PCa variants for the FRR and heritability calculations [3] , [11] . For these analyses, we used conditional estimates from fitting a single model with all variants in the OncoArray dataset for regions with multiple variants and the overall marginal meta-analysis results from Schumacher et al. [3] for regions with a single variant. To correct for potential bias in effect estimation of newly discovered variants, we implemented a Bayesian version of the weighted correction [32] , which incorporates the uncertainty in the effect estimate into the final estimates of the bias-corrected ORs, 95%CIs and the corresponding calculations of percent FRR explained. JAM analysis To confirm the stepwise results and identify candidate variants for potential functional follow-up, we used a second fine-mapping approach, JAM (Joint Analysis of Marginal summary statistics) [12] . JAM is a multivariate Bayesian variable selection framework that uses GWAS summary statistics to identify the most likely number of independent associations within a locus and define credible sets of variants driving those associations. JAM was applied to summary statistics from the meta-analysis results using LD estimated from imputed individual level data from 20,000 cases and 20,000 controls randomly selected from the OncoArray sub-study. LD pruning was performed using Priority Pruner ( http://prioritypruner.sourceforge.net/ ) on the 2772 marginally associated variants at r 2 = 0.9, resulting in 825 tag variants analyzed in four independent JAM runs with varying starting seeds. Credible sets were determined as the tag variants that were selected in the top models that summed to a specific cumulative posterior probability in all four of the independent JAM runs, plus their designated high LD proxy variants from the pruning step. Functional annotation Variants in the 95% credible set ( n = 50) plus variants correlated at r 2 > 0.9 with those in the credible set ( n = 174) were annotated for putative evidence of biological functionality using publicly available datasets as described by Dadaev et al. [11] . Briefly, variants were annotated for proximity to gene (GENCODEv19), miRNA transcripts (miRBase release 20), evolutionary constraint (according to GERP++, SiPhy and PhastCons algorithms), likelihood of pathogenicity (CADDv1.3) and overlap with prospective regulatory elements in prostate-specific datasets (DNaseI hypersensitivity sites, H3K27Ac, H3K27me3 and H3K4me3 histone modifications, and for AR, CTCF, ERG, FOXA1, GABPA, GATA2, HOXB13, and NKX3.1 transcription factor binding sites) in a mixture of LNCaP, PC-3, PrEC, RWPE1, and VCaP cell lines and human prostate tumor tissues downloaded from the Cistrome Data Browser ( http://cistrome.org/db/ ). The chromatin state in which each variant resides was assessed using ChromHMM annotations from two prostate cell lines (PrEC and PC3). Cis-gene regulation was evaluated using 359 prostate adenoma cases from The Cancer Genome Atlas (TCGA PRAD; https://gdc-portal.nci.nih.gov ) that passed QC [11] . The eQTL analysis was performed using FastQTL with 1000 permutations for each gene within a 1Mb window. We then used the method by Nica et al. [33] that integrates eQTLs and GWAS results in order to reveal the subset of association signals that are due to cis eQTLs. For each significant eQTL, we added the candidate variant to the linear regression model to assess if the inclusion better explains the change in expression of the gene. We retrieved the p -value of the model, assigning p-value of 1 if the eQTL and variant are the same. Then we ranked the p-values in descending order for each eQTL, and finally calculated the colocalization score for each pair of eQTL and variants. In general, if an eQTL and candidate variant represent the same signal, this will be reflected by the variant having a high p-value, a low rank and consequently a high colocalization score.